Imaging local electronic corrugations and doped regions in graphene Electronic structure heterogeneities are ubiquitous in two-dimensional graphene and profoundly impact the transport properties of this material. Here we show the mapping of discrete electronic domains within a single graphene sheet using scanning transmission X-ray microscopy in conjunction with ab initio density functional theory calculations. Scanning transmission X-ray microscopy imaging provides a wealth of detail regarding the extent to which the unoccupied levels of graphene are modified by corrugation, doping and adventitious impurities, as a result of synthesis and processing. Local electronic corrugations, visualized as distortions of the π*cloud, have been imaged alongside inhomogeneously doped regions characterized by distinctive spectral signatures of altered unoccupied density of states. The combination of density functional theory calculations, scanning transmission X-ray microscopy imaging, and in situ near-edge X-ray absorption fine structure spectroscopy experiments also provide resolution of a longstanding debate in the literature regarding the spectral assignments of pre-edge and interlayer states. The demonstration of remarkable transport phenomena in graphene, a two-dimensional hexagonal lattice of carbon atoms, in 2004 by Geim and Novoselov, has inspired a paradigm shift in viewing electronic structure and electron–phonon coupling for condensed matter systems exhibiting aspects of quantum relativistic phenomena [1] . Some notable features of graphene that make it a remarkable model system for condensed matter physics and solid state chemistry include massive room-temperature carrier mobilities, ballistic conduction across micrometer lengths, and the anomalous quantum Hall effect [2] , [3] , [4] . These remarkable properties are a consequence of the distinctive band structure of graphene. Electronic band energies follow linear dispersion relations with respect to electron momentum in the vicinity of two symmetry-inequivalent points, K and K ′, in the 2D Brillouin zone. The ground state Fermi level is located at these so-called Dirac points-the conical intersection of these linear bands. Thus, electrons propagating through the conduction band encounter no potential barriers and essentially behave as itinerant massless Dirac fermions, the crux of most novel electronic phenomena observed in this unwonted system [5] . The range of novel observed phenomena is expected to expand, predicated on increased success with chemical vapour deposition growth of large-area graphene sheets and improved crystalline quality. Nevertheless, several aspects of the fundamental electronic structure of graphene remain underexplored, particularly with reference to local electronic domains that are induced by inevitable rippling or doping of discrete regions. Knowledge of such phenomena, and understanding band structure alterations originating from the formation of localized electronic domains are imperative to facilitate the integration of graphene within commercial electronics, for applications ranging from interconnects to high electron mobility transistors [1] , [6] , [7] , [8] . The rippling and doping of discrete regions of the graphene lattice is a consequence of the one-atom-thick 2D nature of this material, which being uniquely composed of atoms that reside entirely on the surface is highly susceptible to interactions at interfaces and the influence of adventitious impurities that can locally perturb the electronic structure [9] , [10] . Doping and adsorbates are somewhat inevitable as a result of typical processing protocols including wet and dry transfer techniques ubiquitous in the transfer of chemical vapour deposition (CVD)-grown graphene; chemical etching required for removal of Si, Cu, and Ni substrates; and solvent washes used to clean residue from graphene surfaces or for lithographic patterning. Near-edge X-ray absorption spectroscopy (XAS) techniques are well established for characterizing element-specific electronic structure with extremely high surface sensitivity, making it an ideal tool for the study of graphene [11] . The peak positions and lineshapes of the observed XAS resonances represent, to first approximation, a replica of the unoccupied atom-projected density of states modified by core–hole interactions. Scanning transmission X-ray microscopy (STXM) involves raster scanning a finely focused soft X-ray beam over the object of interest to obtain an exquisitely detailed spatial map of the unoccupied density of states (UDOS), thereby providing a means to directly image electronic structure. The rigorous comparisons of experimental STXM and near-edge X-ray absorption fine structure (NEXAFS) data with ab-initio X-ray absorption calculations that take into account core–hole interactions provides an unprecedented insight into the electronic structure of graphene. The theoretical spectra were computed using the Fermi's Golden Rule expression for the X-ray absorption cross-section (σ), defining the probability of exciting a core electron from an initial state, ψ i to a final state, ψ f by X-ray photons: where α 0 is the fine structure constant and ℏ ω is the photon absorption energy, which should equal E f −E i , the energy difference between initial and final states. The matrix elements, , are evaluated with respect to the product of the polarization direction of the photon electric field, εε^ , and the single-electron position operator, r , for effective single-particle states derived from density functional theory (DFT) calculations and accurate up to a factor S ≤ 1 , approximately constant for all transitions [12] , [13] , [14] . Therefore, the X-ray absorption cross-section is directly related to the energy density of the final states, accounting for the close correlation between STXM and NEXAFS data and the UDOS. Geometry optimization and band-structure calculations were performed using the Quantum ESPRESSO suite of computational codes [15] . The STXM and NEXAFS methodologies described here are not intended to supplant standard characterization methods; instead, the approaches used here provide necessary fundamental understanding by discriminating between electronic defects that are otherwise indistinguishable and enabling unprecedented direct imaging of the prevalence of electronic structure inhomogeneities in graphene. The possible imperfections examined in this submission are corrugation, doping, and surface adsorbates, but edge effects, layer–layer stacking, and missing atoms have also been recently shown to distort the band structure [16] . Here we present the direct experimental mapping (with ∼ 40 nm spatial resolution) of discrete electronic domains within a single graphene sheet, and further use DFT calculations to elucidate the electronic structure of graphene in unprecedented detail; thus resolving several controversies that have recently emerged regarding the assignment of features in the X-ray absorption fine structure spectra of graphene [17] , [18] , [19] . STXM mapping of the electronic structure of graphene Figures 1a and 2a show integrated C K-edge (280–320 eV) STXM images of two distinct single-layered graphene samples, wherein distinctive regions with apparently different optical densities have been demarcated. Mapping of spectral features was accomplished using aXis2000 (ref. 20 ). The transmission data is converted to optical density (OD) by I / I 0 where I , the intensity transmitted is divided by I 0, the background signal, which are simultaneously measured; thus, both the sample ( I ) and an empty region ( I 0 ) must be within the raster scanned region to acquire spectra. Each feature is a summation of 0.3 eV energy step scans through regions of interest. The stack corresponding to the number of spectral scans is then averaged by the number of steps and then divided by the scan image at 320 eV to normalize against the amount of carbon. 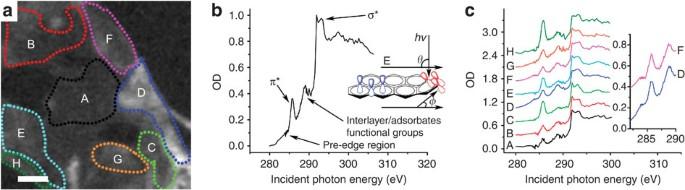Figure 1: STXM mapping of the electronic structure of graphene. STXM images and data of CVD grown SLG on Cu after wet etching in HNO3and transfer. (a) Transmission mode data is converted to OD byI/I0, whereI0is measured in an empty scan region; summation of 0.3 eV energy steps is normalized to carbon at 320 eV. Corresponding white intensity describes the thickness and morphology of the graphene sheet. The scale bar is 1 μm and the total distance across the image is 4 μm. (b) Integrated C K-edge spectrum of entire image in (a). The electromagnetic field vector (E) and incident X-ray photon energy (hν) are at angle (θ). The angular difference between the pristine basal plane (blue π orbitals) and the asperity (red π orbitals) represent a degree of corrugation (φ) of a rippled graphene sheet. (c) Isolated C K-edge spectra of each region displayed in (a), where spectra D and F displayed in the inset have the most prominent pre-edge features. The pre-edge feature is further clearly discernible inFigures 2and3. Figure 1: STXM mapping of the electronic structure of graphene. STXM images and data of CVD grown SLG on Cu after wet etching in HNO 3 and transfer. ( a ) Transmission mode data is converted to OD by I/I 0 , where I 0 is measured in an empty scan region; summation of 0.3 eV energy steps is normalized to carbon at 320 eV. Corresponding white intensity describes the thickness and morphology of the graphene sheet. The scale bar is 1 μm and the total distance across the image is 4 μm. ( b ) Integrated C K-edge spectrum of entire image in ( a ). The electromagnetic field vector (E) and incident X-ray photon energy ( hν ) are at angle ( θ ). The angular difference between the pristine basal plane (blue π orbitals) and the asperity (red π orbitals) represent a degree of corrugation ( φ ) of a rippled graphene sheet. ( c ) Isolated C K-edge spectra of each region displayed in ( a ), where spectra D and F displayed in the inset have the most prominent pre-edge features. The pre-edge feature is further clearly discernible in Figures 2 and 3 . 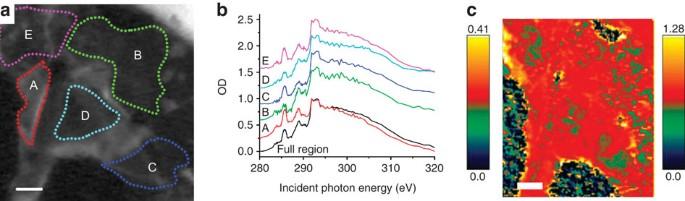Figure 2: Mapping the electronic corrugations of graphene. STXM images of CVD-grown SLG on Cu after wet etching in HNO3and transfer. (a) Transmission mode data is converted to OD byI/I0, whereI0is measured in an empty scan region. The white scale bar is 1 μm with a total distance across the entire image of 4 μm. (b) Integrated C K-edge spectra of isolated regions depicted in (a). False colour images displaying (c) the π*resonance in the proximity of 285.5 eV. The colour scale on the left represents the absolute OD, whereas the scale to the right denotes the normalized OD. Note the pre-edge intensity seen in spectra/regions B and E and the intense white region in the upper right corner, representative of a graphitic flake. Full size image Figure 2: Mapping the electronic corrugations of graphene. STXM images of CVD-grown SLG on Cu after wet etching in HNO 3 and transfer. ( a ) Transmission mode data is converted to OD by I / I 0 , where I 0 is measured in an empty scan region. The white scale bar is 1 μm with a total distance across the entire image of 4 μm. ( b ) Integrated C K-edge spectra of isolated regions depicted in ( a ). False colour images displaying ( c ) the π*resonance in the proximity of 285.5 eV. The colour scale on the left represents the absolute OD, whereas the scale to the right denotes the normalized OD. Note the pre-edge intensity seen in spectra/regions B and E and the intense white region in the upper right corner, representative of a graphitic flake. Full size image Graphene was grown in a home-built CVD reactor at ambient pressure and at ∼ 1,000 °C using a mixture of Ar, H 2 and CH 4 gases, as further detailed in the Methods section. Subsequently, the graphene samples were transferred to a Cu TEM (transmission electron microscopy) grid for analysis by STXM. In Figure 1 , the normalized optical density in region A is single-layered graphene, whereas the corresponding brighter regions are folded regions with multiple single-layered graphene layers. Figures 1 shows the composite integrated spectrum measured for the graphene sheet, along with assignments to transitions to specific unoccupied states above the Fermi level such as the π*and σ*states along with putative interlayer/functionality and pre-edge regions: the latter two assignments being particularly contentious. 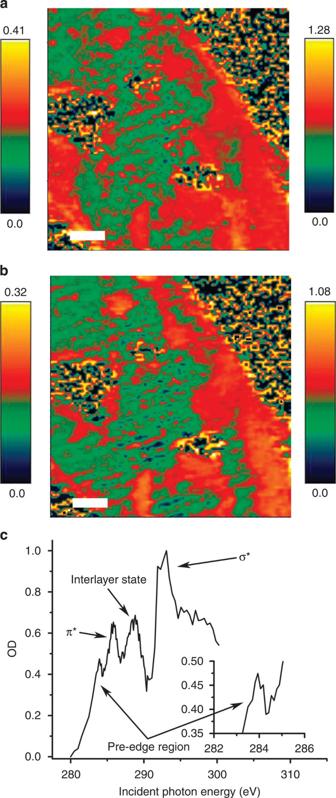Figure 3: Mapping doped regions and corrugations of graphene. False colour images displaying (a) π*at 285.5 eV and (b) pre-edge at 283.7 eV, where each image shows prominent C K-edge resonances. Colour scales on the left represent absolute OD values, and to the right reflect the normalized OD, referenced to the carbon signal at 320 eV. The scale bar corresponds to 1 μm with a total distance across the image of 4 μm. The pre-edge peak is prominent in (c), where only high (red–yellow) OD regions in (b) were selected for the spectrum. The pre-edge feature is more prominently visible within specific domains for the graphene sheet shown in Figure 3 . Figure 3: Mapping doped regions and corrugations of graphene. False colour images displaying ( a ) π*at 285.5 eV and ( b ) pre-edge at 283.7 eV, where each image shows prominent C K-edge resonances. Colour scales on the left represent absolute OD values, and to the right reflect the normalized OD, referenced to the carbon signal at 320 eV. The scale bar corresponds to 1 μm with a total distance across the image of 4 μm. The pre-edge peak is prominent in ( c ), where only high (red–yellow) OD regions in ( b ) were selected for the spectrum. Full size image The spectra for the individual demarcated regions, as shown in Figures 1 and 2, delineate substantiative differences in the relative intensities of π* and pre-edge spectral features across the different regions. The modulations captured for π*peak intensities across the graphene sheet are due to the presence of geometric corrugations in the material. As STXM data has been acquired at normal incidence using polarized soft X-ray radiation, based on dipole selection rules, an orbital with perpendicularly symmetric orientation to the basal plane of graphene (π*) should not be resonant; this is a result of the electric field vector of the incident beam being coincident with the nodal plane, depicted by the blue (perpendicular) and red (tilted) π* orbitals in Figure 1b . Consequently, increased π*intensities relative to the σ* can be correlated to electronic corrugations or asperities that are aligned with the electric field vector of the incident radiation, according to angle φ depicted in Figure 1b (see Supplementary Equation S1 , see Supplementary Information for discussion), where the electronic corrugations in Regions A–H correspond to φ values of π/6, 2π/9, π/4, π/4, π/4, π/4, 2π/7 and 2π/7, respectively. The pronounced π*feature is apparent for Region H, corresponding to a distinctive fold or ripple in the structure, whereas Region A has a much attenuated π*intensity, suggestive of a flatter graphene domain. Residual π*intensity observed even for this domain is indicative of a rippled topography. The distinctive spectra indicated in Figure 1c for the different topographical regions thus indicate the formation of electronic domains with modified corrugations. Figure 2 illustrates STXM data acquired for a similarly corrugated graphene sheet with distinctive electronic domains; additionally, the top-right corner depicts an intense π*contribution from a separate few-layer graphene fragment. An analogous description of corrugation and rippling could be extrapolated from the demarcated regions in Figure 2 . In Figure 3, a false colour map of Figure 1a for the π*peak centred at 285.5 eV is presented, clearly identifying the presence of ripples and folds across the sample (visualized as red and yellow regions). Although the π*features can easily be correlated to asperities that induce electronic corrugations ( Figure 2c ), the pre-edge feature plotted in Figure 3b is not readily correlated to such topographical features. The inset in Figure 1c shows spectra D and F that have the most pronounced pre-edge features, but interestingly each region has dissimilar topography, suggesting that variations in intensity of this feature are not a result of dipolar orientation. The corresponding spectra for another sheet of graphene shown in Figure 2 are characterized by stronger contributions from the pre-edge features, again localized within distinctive domains. Ab-initio modelling of graphene spectral signatures To definitively evaluate current understanding of the assignment of graphene X-ray absorption spectral features and to resolve a longstanding debate, we performed ab-initio XAS calculations that explicitly take into account the core–hole interactions. 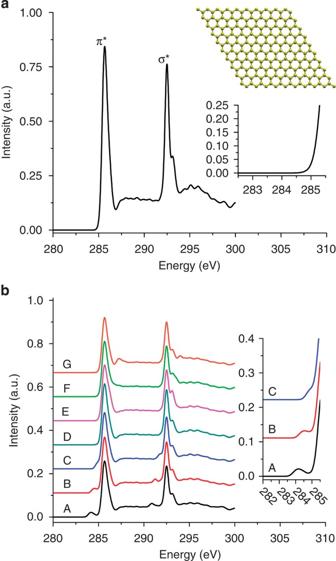Figure 4: Modelling the XAS Spectral Signatures of Graphene and Doped Graphene. Ab-initioFCH-XAS calculations of a single layer of carbon atoms (200-atom periodic cell) depicted at magic incidence (54.7°) for ease of comparison with NEXAFS data. (a) Calculated C K-edge spectrum of a periodic pristine sheet, the energy has been calibrated to the sharp π*NEXAFS feature. The inset has no discernible features in the pre-edge energy region. (b) Delocalized ionizations of the 200-atom sheet, where spectra A-C (−3, −2, −1) and E-F (+1, +2, +3) are charged surfaces and spectrum D is neutral; charges (−1, −2, −3) are in units of e. 10% of the ionized spectra are summed with 90% of the neutral spectra to represent a 10% dopant level. In Figure 4a , we show a C-K edge spectrum calculated for a 200 atom hexagonal supercell of graphene ( a= 2.420 nm) under periodic boundary conditions with no edge states. The spectrum has been modelled with a pseudopotential approximation previously reported by some of the authors [14] . The X-ray excited atom is derived from a carbon pseudopotential with one electron removed from the 1 s level. The unoccupied electronic levels are generated within DFT from a self-consistent potential that incorporates the perturbation of the core–hole pseudopotential on just one C atom in this large supercell. We use the Perdew-Burke-Ernzerhof [21] form for the exchange–correlation potential within the generalized-gradient approximation. For the excited state, we have determined that the full-core-hole (FCH) approximation more accurately captures the charge density of the lowest-energy core–hole excited state (at absorption onset) in the extended graphene system. The FCH approximation includes the core–hole perturbation without explicit inclusion of the lowest-energy excited electron within the supercell. The first available unoccupied states in graphene are completely delocalized π*states, which do not become significantly localized due to the core–hole binding energy. For our supercell sizes, under periodic boundary conditions, the use of the excited electron and core–hole (XCH) approximation would place an additional electron in each supercell and would constitute an unphysically large doping concentration (that is, number of free carriers at the Fermi level), with a noticeable spurious impact on the core-excited density of states and associated X-ray absorption spectrum. This is contrary to the more common application of the XCH approximation to bound excitons in the X-ray excitations of molecules and molecular condensed phases [14] , [22] , [23] . Figure 4: Modelling the XAS Spectral Signatures of Graphene and Doped Graphene. Ab-initio FCH-XAS calculations of a single layer of carbon atoms (200-atom periodic cell) depicted at magic incidence (54.7°) for ease of comparison with NEXAFS data. ( a ) Calculated C K-edge spectrum of a periodic pristine sheet, the energy has been calibrated to the sharp π*NEXAFS feature. The inset has no discernible features in the pre-edge energy region. ( b ) Delocalized ionizations of the 200-atom sheet, where spectra A-C (−3, −2, −1) and E-F (+1, +2, +3) are charged surfaces and spectrum D is neutral; charges (−1, −2, −3) are in units of e. 10% of the ionized spectra are summed with 90% of the neutral spectra to represent a 10% dopant level. Full size image The assignment of the area denoted as interlayer states and the distinctive pre-edge features noted for some of the domains in Figures 1c and 2b have been the topic of much recent contention for single-layered graphene (SLG) [16] , [17] , [18] , [19] . The latter resonance has been ascribed to a peculiarity in the band structure of single-layered graphene. Pacilé et al . proposed that the pre-edge resonance (283.7 eV) arises from a UDOS splitting of the π*feature along the high-symmetry direction in momentum space that is peculiar to single-layered graphene [24] ; although, most notably, they referenced a ground-state band structure calculation [25] . Note that the impact of the C 1 s core–hole excitation on the density of states is significant enough to modify the local band structure and this is specifically what is probed in X-ray absorption. Most recently, in an all-electron DFT calculation, Hua et al ., have refuted this assignment and have instead ascribed this feature to missing carbon atoms and edge effects that perturb the UDOS [16] . Notwithstanding, given the quick decay of the distinctive signal away from the edge, in principle, a far smaller spot size would be required to sample enough edge atoms to produce these features as compared with the current spatial resolution of STXM and PEEM (photoemission electron microscopy) techniques (on the order of 40 nm; pixel size is ∼ 0.016 μm 2 ). Our DFT calculations for hydride-terminated graphene fragments further corroborate that the distinctive spectral feature of edge carbon atoms (a splitting of the π*resonance) is lost, and the 'bulk' electronic structure is recovered even for atoms in close proximity to the edge, suggesting that highly localized edge states will not be detectable by STXM for samples with the dimensions imaged here (such states may perhaps be observable for ultra-small nanoribbons with a much greater contribution from edge states). The assignment of the interlayer state (287–289 eV) has also been contentious and alternative descriptions ascribe these peaks to residual functionalization, typically C–O or C–H bonding [18] , [26] surface contamination or as a dispersion of three-dimensional unoccupied bands in graphite [27] Graphite itself has a prominent interlayer state that has been observed using NEXAFS spectroscopy in three distinctive modes: electron yield, fluorescence yield and transmission yield [28] . The XAS spectrum computed by ab-initio methods depicted in Figure 4a shows no pre-edge or interlayer state. The spectra in Figure 4b were aligned with reference to spectrum D (neutral), which was calibrated to 285.7 eV (NEXAFS) by summing the difference between the Fermi energies and the ground state and excited state total energies, accounting for the chemical shift [29] The inset has no characteristic pre-edge features suggesting that such an absorption feature is not an intrinsic characteristic of SLG. An alternative scenario that would explain the seemingly random occurrence of these peaks in distinctive domains of the graphene sheet, as indicated in Figures 1 , 2 and 3 , is to consider locally doped regions that may well result from interactions with oxidizing and reducing agents during processing (acid treatment and etching for this specific example). Figure 4b shows the summation of the spectrum depicted in Figure 4a for undoped graphene (90% contribution) with spectra similarly calculated for electron or hole dopants considered to be delocalized over the entire supercell (10% percent contribution). For doped graphene, the spectra are very similar to the undoped state but the peak positions are rigidly shifted along the energy axis. XAS edge energies are sensitive to oxidation state changes and charge transfer, according to Kunzl's law wherein a positive or negative oxidation state will blue- or red-shift the Fermi energy (E f ), respectively [30] . From A–G, the spectra correspond to different ionization levels representing the addition of electrons or holes to the supercell. In this case, one, two or three electrons or holes were added to a 2.420 nm graphene supercell corresponding to delocalized charge densities of 6.6×10 −6 , 1.32×10 −5 and 1.98×10 −5 C cm −2 . Remarkably, the modest 10% doped contribution invoked here very successfully captures the pre-edge peaks noted in Figure 1c and reported by Pacilé et al . A pre-edge peak ascribed to dopant-induced states has indeed been observed for graphite and carbon nanotubes intercalated with FeCl 3 (refs 10 , 31 , 32 ), where again it is clear that the feature arises from extraneous modulation of the band structure rather than an intrinsic peculiarity. The inset to Figure 4 shows the pre-edge feature shifts energetically according to the charge (-3:A, -2:B, -1:C), which could potentially arise from a combination of HNO 3 , HF, FeCl 3 , Fe(NO 3 ) 3 , metal-hydroxides or analogous charged species used for convent i onal lithographic processing and transfer of graphene. 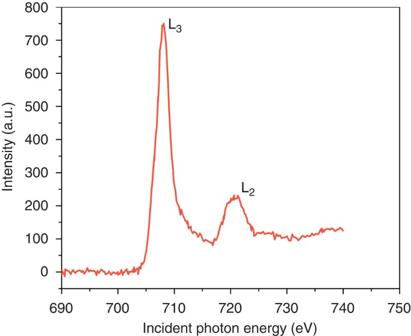Figure 5: Detection of Fe on Graphene. NEXAFS Fe L-edge spectrum of SLG on SiO2, after transfer. Detectable concentrations of Fe on SLG are noted due to etchants, FeCl3or Fe(NO3)3, after processing and transfer. Figure 5 depicts Fe L-edge spectrum of graphene that has been transferred after etching of the underlying Cu substrate with aqueous Fe 3+ . The spectrum shows prominent L 3 and L 2 resonances, clearly verifying the presence of adsorbed iron-species remnant on the graphene sample. Therefore, electron excitations that induce charge transfer can potentially create a pre-edge feature by simultaneously sampling an inhomogeneous distribution of discrete doped and undoped regions with distinct chemical potentials, represented here in a 1-to-9 ratio as an illustrative example. Note that the effect of such delocalized doping in graphene is very distinctive from substitutional doping with nitrogen or boron, which leads to distinctive spectral signatures from α and β sublattices and tends to be localized in the proximity of the incorporated point defect. Figure 5: Detection of Fe on Graphene. NEXAFS Fe L-edge spectrum of SLG on SiO 2 , after transfer. Detectable concentrations of Fe on SLG are noted due to etchants, FeCl 3 or Fe(NO 3 ) 3 , after processing and transfer. Full size image Another alternative explanation that cannot be ruled out, is that doping shifts the Dirac point in graphene and uncovers features of the occupied density of states that are then visualized as shoulders to the π*feature. The formation of electronic corrugations may very well limit doping to specific regions, accounting for the stronger intensity of the pre-edge feature only within certain regions of the graphene sheet ( Fig. 3b ). Indeed, electron–hole puddles probably derived from analogous adventitious dopants are known to give rise to electrostatic fluctuations in graphene, acting as Coulomb scatterers, as has been evidenced in some elegant low-temperature single-electron transistor measurements [33] . The 'Interlayer' state? Figure 4a also suggests that the putative 'interlayer state' ascribed by Pacilé et al ., as the intermediate between the π*and the σ*bands, is not an intrinsic feature of SLG [17] , [18] , [19] . To arrive at a better understanding of the origin of these features, we have annealed graphene samples in situ . 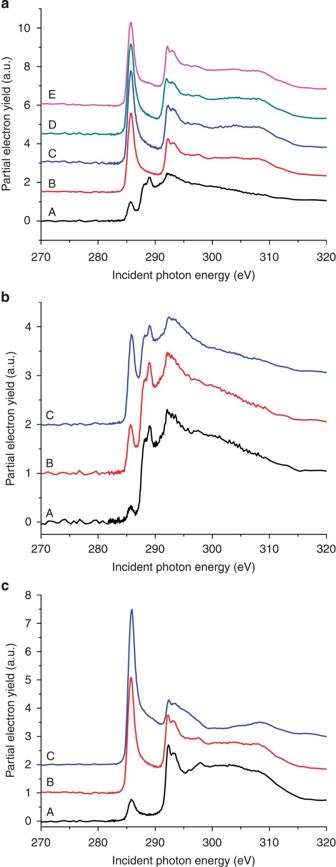Figure 6:In- situannealing of graphene monitored by NEXAFS spectroscopy. (a)In situheating of CVD-grown SLG on Cu, where A–D were acquired at 30, 150, 300, 450 °C, respectively. The C K-edge spectra were acquired under ultra high vacuum (UHV) and at a magic angle of incidence (54.7°). Spectra E was acquired after the sample was heated to 650 °C and cooled back to room temperature within the UHV chamber. The interlayer/adsorbate/functional group region has no resonaces after annealing to 150 °C. (b) Three angles A–C (85°, 54.7° and 25°) at room temperature and (c) at 150 °C, as measured at the C K-edge. Figure 6 depict NEXAFS spectra acquired during a heating cycle for graphene grown on a Cu substrate at magic angle incidence; angle-resolved NEXAFS data is also presented suggesting that this spectral feature does not substantially exhibit polarization dependence. Remarkably, after in situ heating to only 150 °C, the purported 'interlayer state' vanishes, suggesting that a better assignment may be to adsorbed impurities. After cooling the sample back to room temperature in vacuuo we see that the intermediate bands do not return, further corroborating that their assignment is to extraneous interactions and not to intrinsic band-structure peculiarities of graphene. Notably, the intermediate peaks are recovered if the graphene sample is exposed to atmospheric conditions for sufficiently long periods of time shown in Supplementary Figure S1 ; possible adsorbates could be CO, CO 2 , and aliphatic alcohols from solution processing of graphene. Notably, no evidence of C–H peaks has been observed in either Raman spectroscopy or Fourier transform infrared spectroscopy measurements ( Supplementary Figs S2 and S3 ) ruling out a substantial contribution from these species. Covalent modification of graphene is possible during acid etching [34] and graphene oxide has characteristic features in this regime arising from carboxylic acid, ketone, epoxide and alcohol moieties (as shown by the spectrum in Supplementary Fig. S4 ). However, defunctionalization at such low temperatures is unlikely for covalently modified functional groups suggesting that the peak is unlikely to be preponderantly of functional group origin [35] . At the same time, contributions from acid-induced functional groups can not be ruled out. In this context, analogous diminution of putative interlayer states has also been noted in measurements of carbon nanotubes upon in situ heating corroborating the assignment of these features to adsorbates [36] . Figure 6: In- situ annealing of graphene monitored by NEXAFS spectroscopy. ( a ) In situ heating of CVD-grown SLG on Cu, where A–D were acquired at 30, 150, 300, 450 °C, respectively. The C K-edge spectra were acquired under ultra high vacuum (UHV) and at a magic angle of incidence (54.7°). Spectra E was acquired after the sample was heated to 650 °C and cooled back to room temperature within the UHV chamber. The interlayer/adsorbate/functional group region has no resonaces after annealing to 150 °C. ( b ) Three angles A–C (85°, 54.7° and 25°) at room temperature and ( c ) at 150 °C, as measured at the C K-edge. Full size image The increased corrugation and rippling of graphene evidenced in Figures 1 , 2 , 3 and arising as a result of typically processing, has tremendous implications for the mobilities of charge carriers. It has been predicted that electrons propagating through graphene are scattered by corrugations and ripples in the graphene sheet through a potential V ( r ) [4] , [37] , that is approximately proportional to the square of the local curvature. In equation (2), α is a constant ( α =10 eVÅ 2 ) that depends on the microscopic details, whereas h ( r ) is the height field that depends on the local curvature R according to: Crumpling of the graphene sheets has an analogous effect on the electron mean-free path as the presence of Coulombic scatterers. A similar dependence has been shown, where charged impurities and ripples have been found, by Katsnelson and Geim, to scatter Dirac fermions in graphene [38] and more recently, extended 1D charge defects were corroborated to scatter carriers through an analogous process [39] . Lee and co-workers recently demonstrated hole mobility values of ∼ 1,630 cm 2 /(V s)±140 cm 2 /(V s) for devices constructed using transferred graphene grown by CVD on either Cu or Ni substrates based on measurements of ∼ 1,600 devices [40] . The measured hole mobility values are more than two orders of magnitude smaller than values obtained for micromechanically cleaved graphene samples on Si/SiO 2 , suggesting that the transfer process has a deleterious impact on the measurements. Based on the significant decrease in anisotropy noted in our optical density map after transfer, it is likely that rippling and corrugation have an important role in suppressing measured charge transfer mobilities by introducing electronic boundaries. There has also been an interest in probing grain boundaries in graphene with dimensions on the order of ∼ 10.0–0.063 μm 2 using high-resolution transmission electron microscopy(HRTEM) and dark field TEM for graphene samples grown via CVD on Cu (refs 41 , 42 ). The discrete domains visualized in Figures 1 , 2 , 3 are essentially correlated to corrugations within discrete graphene sheets, although the top-right of Figure 2a demonstrates a distinctive separate few-layered graphene fragment characterized by a highly intense bright region. Grain boundaries are likely to be electronically manifested in the form of a modified angle of the π*UDOS presented to the incident beam and, consequently, are a probable origin of the electronic corrugations visualized here, although a more detailed correlation of the atomic and electronic structure is required to suggest the spectral signature of a graphene grain boundary. Notably, a 'high-angle' grain boundary would be most likely to have an electronic structure signature detectable by STXM or NEXAFS. Thus, combining ab-initio DFT calculations with in situ NEXAFS and localized STXM measurements allows for a rigorous exploration of the localized electronic structure of graphene. The π*electronic spectrum has been mapped with respect to the intensity of the optical density and spectral features to determine the extent of corrugating rippling. Evaluating such corrugation, and associated band structure changes with formation of 'electronic grain boundaries' is imperative for fundamental understanding of phenomena measured for large-area graphene samples as well as for their technological implementation within device architectures requiring high mobilities. DFT calculations have also enabled unprecedented insight into the influence of doping and surface contamination in altering the UDOS. This allows us to settle an ongoing debate in the literature regarding the origin of the pre-edge feature and interlayer states. The pre-edge feature in particular has been mapped and is observed to be localized within specific domains that are susceptible to doping, but somewhat limited by corrugation. At the same time, we demonstrate that graphene is impacted by environmental contamination due to adsorption of impurities under ambient conditions or during solution processing. The localized electronic structure ideas reported here also pave the way for understanding discrete electronic domains within other Dirac point materials as well as graphene incorporating substitutional dopants. Future work will focus on NEXAFS studies of graphene metal-interfaces and chemical dopants. Sample preparation Graphene was grown by CVD onto Cu and Ni substrates as described previously [43] , [44] , [45] ; for STXM the samples were transferred onto a 300 mesh Cu TEM grid subsequent to release from the substrate by etching with a solution of 5:1 DI:HNO 3 (ref. 40 ). Supplementary Figure S5 ( Supplementary Information ) shows a transmission electron microscopy image and selected area electron diffraction pattern corroborating the growth of single-layered graphene transferred onto a 400 mesh SiO/Cu TEM grid by an analogous etching process. Supplementary Figure S2 depicts Raman spectra of graphene grown on Cu and Ni substrates; Supplementary Figure S6 shows the corresponding NEXAFS spectra. CVD growth on Cu provides better homogeneity and control over the number of graphene layers and consequently these samples have been analysed further in the STXM measurements. As we have shown in previous work, the π*feature of graphene on metal foil substrates is split because of the substrate hybridization likely with Cu/Ni d z 2 orbitals [9] . The strength of such interfacial bonding, as evidenced by splitting of the π*feature in Supplementary Figure S6 ( Supplementary Information ), is greater for the graphene/Ni interface as compared with graphene grown on Cu. The peak shifts of the 2D Raman band can be related to its origin from a double-resonance phonon scattering process; SLG has no graphene layer–layer interaction and the intervalley scattering of the two phonons are degenerate, whereas the number of non-degenerate dispersions increases in bilayered graphene (increasing the number of K points and thus the number of possible scattering events) with the overall consequence of shifting and broadening of the 2D resonance [46] , [47] . Notably, charge transfer interactions with the underlying substrate can also shift the Raman modes of graphene. Scanning transmission X-ray microscopy STXM data was collected at beamline 10ID-1 of the Canadian Light Source. The STXM end-station has an elliptically polarized undulator source with a slitless entrance-plane grating monochromator. Incoming X-rays are focused using a Fresnel lens zone plate including an order-sorting aperture to remove unwanted diffraction orders. The optics design allows for high flux in transmission geometry and operating spatial resolutions of ∼ 40 nm (30 nm focal spot size). Sampling areas are raster scanned through the focal point of the X-ray beam, and transmitted beam intensities are measured at the detector pixels. Energy scans were performed stepwise through regions of interest (130–1,500 eV) with typical resolving power (Δ E / E ) of 2×10 −4 . Near edge X-ray absorption fine structure spectroscopy Carbon K-edge NEXAFS heating experiments were performed at National Institute of Standards and Technology (NIST) beamline U7A of the National Synchrotron Light Source at Brookhaven National Laboratory. A toroidal spherical grating monochromator with 600 lines per mm was used to acquire the C K -edge data yielding an energy resolution of approximately 0.1 eV. The slits were set to 30 μm by 30 μm. The spectra were acquired in partial electron yield mode (PEY) with a channeltron electron multiplier detector with an entrance grid bias set to −150 V to enhance surface sensitivity. A charge compensating electron charge gun was used to remove the effects of charging. The partial electron yield mode signals were normalized using the incident beam intensity obtained from the photoemission yield of a freshly evaporated Au grid with 90% transmittance placed along the path of the incident X-rays. The C K-edge spectra were calibrated to an amorphous carbon mesh with a π*transition at 285.1 eV. How to cite this article: Schultz, B. J. et al . Imaging local electronic corrugations and doped regions in graphene. Nat. Commun. 2:372 doi: 10.1038/ncomms1376 (2011).